Changing cell behaviours during beetle embryogenesis correlates with slowing of segmentation Segmented animals are found in major clades as phylogenetically distant as vertebrates and arthropods. Typically, segments form sequentially in what has been thought to be a regular process, relying on a segmentation clock to pattern budding segments and posterior mitosis to generate axial elongation. Here we show that segmentation in Tribolium has phases of variable periodicity during which segments are added at different rates. Furthermore, elongation during a period of rapid posterior segment addition is driven by high rates of cell rearrangement, demonstrated by differential fates of marked anterior and posterior blastoderm cells. A computational model of this period successfully reproduces elongation through cell rearrangement in the absence of cell division. Unlike current models of steady-state sequential segmentation and elongation from a proliferative growth zone, our results indicate that cell behaviours are dynamic and variable, corresponding to differences in segmentation rate and giving rise to morphologically distinct regions of the embryo. Bodies built from repeated parts, that is, segmented body plans, are found in three major metazoan taxa—vertebrates, arthropods and lophotrochozoans—and account for an enormous number of extant species. Most of these species develop their segments through a process of sequential budding from the posterior during embryogenesis. Although segment formation was once assumed to be distinct between major taxa, some aspects now appear similar. Sequential segmentation has been studied most extensively in vertebrates, where it relies on regulatory interactions between a segmentation clock that oscillates in the posterior growth zone and a posteriorly moving wavefront that stabilizes the readout of the clock to produce segments [1] , [2] , [3] . The spatial periodic pattern of segmentation is derived from the temporal periodic pattern of oscillating gene expression (the ‘segmentation clock’) in the growth zone [4] . The time to form a segment is species specific [5] , varying from 30 min in zebrafish to 120 min in mouse, but within an individual is relatively constant throughout segmentation and matches the period of each species’ segmentation clock. Typically if variation exists in segment period, it is simply a gradual decrease in segmentation rate as segmentation ‘winds down’ in the posterior of the embryo [6] or a brief initial period of rapid addition prior to a more regular rate [7] . A clock mechanism for regulating segmentation has recently been extended to sequentially segmenting arthropods [8] , [9] , [10] , [11] , [12] , [13] . Support for a clock includes a clear demonstration of molecular oscillations in the flour beetle, Trobolium casteneum [14] . However, species-specific rates of segment addition or variations in those rates are not well-characterized among arthropods, with a few exceptions [15] , [16] . Sequential patterning of segments depends critically on posterior elongation of the growing embryo. In vertebrates, where segments are produced from mesenchymal cells in the presomitic mesoderm, both segmentation and axial elongation are affected by the roles of an FGF8 gradient as a segmentation wavefront and a mediator of cell motility in the presomitic mesoderm [17] . Elongation and its connection to segmentation are less well-characterized in arthropods, whose segments are initially generated within the embryonic epithelium. In the model arthropod, Drosophila , segments are patterned nearly simultaneously in the blastoderm before the embryos elongate. Elongation is achieved through a combination of oriented cell divisions, changes in cell shape and cell intercalation [18] , [19] , [20] , [21] , [22] . This mode of segmentation is a derived condition within arthropods. The vast majority of arthropods elongate from a posterior region, the so-called growth zone [23] , [24] . As the name implies, elongation in the growth zone has been traditionally assumed to be due to high rates of cell division in the posterior [25] , [26] , [27] , [28] . However, other cellular behaviours—cell migration, cell rearrangements, cell shape change—could be used singly or in combination [29] , [30] , [31] , [32] , [33] , [34] . Actual mechanisms of elongation remain poorly described for most arthropods (with the exception of malacostracan crustaceans, which elongate using posterior stem cells [35] , [36] and the centipede Strigamia maritima , which recruits existing tissue to the elongating germ band [37] ). Even in the best-studied sequentially segmenting arthropod, Tribolium , little is known about the cellular processes that lengthen the embryo. Relatively high cell proliferation has been observed in at least one developmental stage of Tribolium [14] , but no one has established a significant role for cell division in elongation [14] , [38] , [39] . By contrast, cell rearrangements have been documented and implicated in elongation: high resolution live imaging in early Tribolium germbands shows that cells in the anterior germband intercalate during elongation [40] and that cells in the early growth zone move posteriorly, towards the midline [14] , [39] , [40] . Nevertheless, these local behaviours have not yet been explicitly linked quantitatively to germband elongation, particularly during later stages. Thus, while growing evidence suggests a requirement for orchestrated cell movements during Tribolium development, no model of intercalary elongation exists and the relative contributions of cell division and cell rearrangement remain unclear. Here we further examine sequential segmentation and germband elongation in Tribolium. We quantify changes in the germband throughout elongation, demonstrating a relatively small increase in overall germband area. We trace clones of cells marked in the blastoderm—in both wild-type and eve knockdown embryos—and confirm that a high degree of cell proliferation is not necessary to drive elongation, at least in the posterior germband in Tribolium . We also demonstrate that posterior blastoderm clones elongate disproportionately compared with anterior clones, and that this spatial variability coincides with temporal variability in segment addition. Segment addition in Tribolium does not have a single periodicity throughout elongation, nor does it decrease monotonically as seen in posterior segmentation in some vertebrates [6] : early segment addition slows significantly and is then followed by a pulse of rapid segment addition midway through germband extension. Moreover, the transition from early segmentation, which gives rise to less elongated clones, to the more rapid later segmentation, which gives rise to more elongated clones, roughly coincides with the morphological thoracic/abdominal transition. This suggests that distinct mechanisms may drive elongation in these two different regions of the embryo, with cell rearrangements being the primary driver of elongation during abdominal segmentation. We support this hypothesis with a computational model of elongation during posterior segmentation that is created solely by cell rearrangements. Segment addition depletes the cells in the growth zone As a first step to understanding elongation during segmentation, we quantified dimensional changes to the germband throughout segment addition, from the time that 1 or 2 gnathal segments are present (11–12 h after egg laying (AEL)) until all 16 post-antennal engrailed (EN) stripes arise. The earliest germband is short and broad and, through a combination of elongation and mesoderm ingression, narrows as segments are added ( Fig. 1 ). During this time, the length of the germband increases more rapidly than the overall area of the germband: there is a 137% increase in germband length ( Fig. 1a ; black) versus only a 41% increase in germband area ( Fig. 1a ; red. Note that these measures do not include cells that have ingressed to form mesoderm). Throughout elongation, segments arise sequentially from the posterior growth zone (defined as the region behind the last EN stripe). As segments are added, the length and area of the posterior growth zone decreases, as does the area of the last newly formed segment ( Fig. 1b,c ). Thus, segment addition depletes the field of cells constituting the growth zone. Indeed, the original growth zone needs to be only ∼ 18% larger to equal the total area of all segments added during extension ( Fig. 1d )—an approximation based on comparison of the average area of the initial growth zone (in germbands with only a mandibular segment) to the total of the average areas of new segments added during germband elongation. Although these calculations subsume the actual complexity of germband elongation to some degree—by wholly ignoring mesodermal ingression—they nonetheless estimate the degree of growth necessary for segmentation. Interestingly, the length of the most recently added segment stays constant over time ( Fig. 1c , black), perhaps reflecting a regulatory process that measures distance from an anterior position or from the immediately anterior segment boundary. A shrinking growth zone and a small increase in overall germband area during segment addition support the hypothesis that a constant high degree of cell proliferation is not required for posterior elongation. 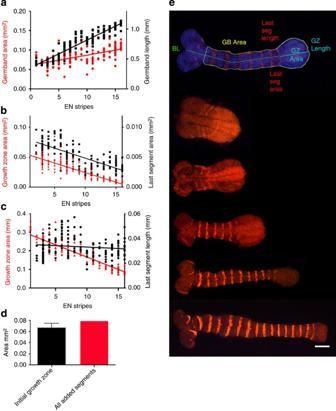Figure 1: Dimensional changes in the elongating germband ofTribolium. (a–c) Quantitative trends in germband dimensions plotted as a function of developmental stage (measured by number of EN stripes, all statistics describe linear regressions). (a) As segments are added inTribolium, the germband increases in length (black,R2=0.89,P<0.0001,n=166) more rapidly than the overall increase in germband area (red,R2=0.34,P<0.0001,n=166). During this time, the growth zone (defined as the region behind the last EN stripe) shrinks both in area (b, red;R2=0.77,P<0.0001,n=163) and anterior/posterior length (c, red,R2=0.81,P<0.0001,n=170). The area of the most recently added segment also decreases during germband elongation (b, black,R2=0.54,P<0.0001,n=163), although its length remains relatively constant (c, black,R2=0.02, not significant). These data are also plotted by developmental stage (Supplementary Fig. 1). (d) The average growth zone area of animals prior to elongation (one EN stripe, black,n=8) needs to be only 18% larger to account for the area at the time of birth of all the segments added during germband extension (red; sum of multiple averages). (e)Triboliumgermbands removed from egg and mounted flat. Top embryo shows measures used in this study (defined in methods); beneath are selected stages stained with EN to show changes in embryo size and shape during germband extension. Scale bar, 100 μm. Figure 1: Dimensional changes in the elongating germband of Tribolium . ( a – c ) Quantitative trends in germband dimensions plotted as a function of developmental stage (measured by number of EN stripes, all statistics describe linear regressions). ( a ) As segments are added in Tribolium , the germband increases in length (black, R 2 =0.89, P <0.0001, n =166) more rapidly than the overall increase in germband area (red, R 2 =0.34, P <0.0001, n =166). During this time, the growth zone (defined as the region behind the last EN stripe) shrinks both in area ( b , red; R 2 =0.77, P <0.0001, n =163) and anterior/posterior length ( c , red, R 2 =0.81, P <0.0001, n =170). The area of the most recently added segment also decreases during germband elongation ( b , black, R 2 =0.54, P <0.0001, n =163), although its length remains relatively constant ( c , black, R 2 =0.02, not significant). These data are also plotted by developmental stage ( Supplementary Fig. 1 ). ( d ) The average growth zone area of animals prior to elongation (one EN stripe, black, n =8) needs to be only 18% larger to account for the area at the time of birth of all the segments added during germband extension (red; sum of multiple averages). ( e ) Tribolium germbands removed from egg and mounted flat. Top embryo shows measures used in this study (defined in methods); beneath are selected stages stained with EN to show changes in embryo size and shape during germband extension. Scale bar, 100 μm. Full size image Anterior and posterior blastoderm clones undergo differential elongation How can this lack of substantial posterior cell division—also reported in Sarazzin et al . [14] —be reconciled with the idea that the posterior region of the blastoderm in sequentially segmenting insects gives rise to a greater proportion of the germband than the anterior [23] ? To explore the relative contributions of cell rearrangement and differential rates of cell division between anterior and posterior blastoderm cells, we traced the fate of small clones made at various positions along the blastoderm to their ultimate positions in the germband. This clonal analysis also allowed us to measure the increase in cell number within each clone over time. As expected, more anterior clones give rise to more anterior segments ( Fig. 2a ; Supplementary Fig. 2 ). However, the number of segments to which a clone contributes depends strikingly on its position along the AP egg axis. Clones posterior to 60% egg length on average give rise to twice the number of segments than do clones that originate between 30 and 60% egg length. Clones made between 60–80% egg length undergo significantly more rearrangement and redistribute into a narrow elongated configuration in the germband ( Fig. 2b,e ). Because all clones divide 2.4 times on average ( Fig. 2c ) regardless of either their initial position in the blastoderm or final position in the germband, positional differences in behaviour cannot be explained by differences in cell division. Interestingly, labelled ectodermal cells in either the anterior or posterior rarely mix with non-labelled cells. Instead, cells within a clone maintain cell contact along the length of the clone. This surprising lack of mixing within a clone and the extreme degree of cellular rearrangement that the clones undergo in the posterior is both novel and unexpected, especially given that clones in the posterior do not divide substantially more than clones in the anterior. The limited amount of post-blastodermal cell division is similar to that observed in ectodermal cells during Drosophila embryogenesis [41] , [42] , [43] and is consistent with our previous measures, suggesting no requirement for a posterior region of rapidly dividing cells generating elongation. The behaviour of these blastoderm clones demonstrates that different degrees of cell rearrangement between anteriorly and posteriorly originating cells (and their progeny), rather than differential division rates, likely account for phenomena that until now have been attributed to a posterior ‘growth zone’ in Tribolium. Notably, the segments spanned by dramatically elongated posterior clones are abdominal segments that are morphologically distinct from the more anterior thoracic segments to which the less elongated clones contribute. 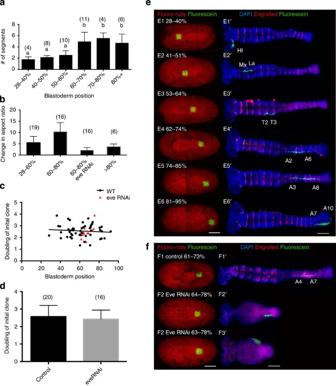Figure 2: Lineage tracing and characterization of blastoderm clones in wild-type andEveRNAi embryos. (a) Number of segments occupied by clones in the extended germband versus original axial blastoderm position. Bars with different letters (a and b) are significantly different. (b) In wild-type embryos, clones at 60–80% egg length (EL) change their aspect ratio more than clones from other positions (analysis of variance,P<0.0001), a result lost ineveRNAi embryos. (c) Doubling of initial clone cell numbers versus original axial blastoderm position show no significant correlation, (linear regression:R2=0.009,P>0.05,n=65). (d) Doubling of 60–80% EL clones in wild-type andeveRNAi embryos do not differ significantly (P>0.05, unpairedt-test). Numbers in parentheses indicate sample sizes for each group ina,bandd. (e) Cell lineage tracing of the blastoderm clones. In blastoderm stage embryos, a small population of the cells is labelled with fluorescein (green, left column). Corresponding later stage embryos (right column) are stained with anti-fluorescein antibody (green), anti-engrailed (red) and DAPI (blue). (E1) 28–40% clone; progeny in the head lobe (Hl). (E2) 41–51% clone; progeny in the maxillary (Mx) and labial (La) segments. (E3) 53–64% clone; progeny in the second and third thoracic segment (T2, T3). (E4) 62–74% clone; progeny in the second to the sixth abdominal segment (A2, A6). (E5) 74–85% clone; progeny in the third to the eighth abdominal segment (A3, A8). (E6) 81–95% clone; progeny in the seventh to the posterior end (A7, A10). Scale bars; 100 μm. (f) Cell lineage tracing of 60–80% EL clones in control andeveRNAi embryos. In the control embryo (F1), the clone undergoes extensive elongation along anteroposterior axis and the descendants occur from the fourth to the seventh abdominal segment (A4, A7). By contrast, in theeveRNAi embryos (F2, F3), clones fail to extend and the descendants remain clustered within the embryos. Scale bar, 100 μm. Figure 2: Lineage tracing and characterization of blastoderm clones in wild-type and Eve RNAi embryos. ( a ) Number of segments occupied by clones in the extended germband versus original axial blastoderm position. Bars with different letters (a and b) are significantly different. ( b ) In wild-type embryos, clones at 60–80% egg length (EL) change their aspect ratio more than clones from other positions (analysis of variance, P <0.0001), a result lost in eve RNAi embryos. ( c ) Doubling of initial clone cell numbers versus original axial blastoderm position show no significant correlation, (linear regression: R 2 =0.009, P >0.05, n =65). ( d ) Doubling of 60–80% EL clones in wild-type and eve RNAi embryos do not differ significantly ( P >0.05, unpaired t -test). Numbers in parentheses indicate sample sizes for each group in a , b and d . ( e ) Cell lineage tracing of the blastoderm clones. In blastoderm stage embryos, a small population of the cells is labelled with fluorescein (green, left column). Corresponding later stage embryos (right column) are stained with anti-fluorescein antibody (green), anti-engrailed (red) and DAPI (blue). (E1) 28–40% clone; progeny in the head lobe (Hl). (E2) 41–51% clone; progeny in the maxillary (Mx) and labial (La) segments. (E3) 53–64% clone; progeny in the second and third thoracic segment (T2, T3). (E4) 62–74% clone; progeny in the second to the sixth abdominal segment (A2, A6). (E5) 74–85% clone; progeny in the third to the eighth abdominal segment (A3, A8). (E6) 81–95% clone; progeny in the seventh to the posterior end (A7, A10). Scale bars; 100 μm. ( f ) Cell lineage tracing of 60–80% EL clones in control and eve RNAi embryos. In the control embryo (F1), the clone undergoes extensive elongation along anteroposterior axis and the descendants occur from the fourth to the seventh abdominal segment (A4, A7). By contrast, in the eve RNAi embryos (F2, F3), clones fail to extend and the descendants remain clustered within the embryos. Scale bar, 100 μm. Full size image Blastoderm clones in ds eve -injected embryos fail to elongate Because the pair-rule gene eve is required for the cell rearrangements that drive germband elongation in Drosophila [19] , we assayed the behaviour of blastoderm clones in embryos injected with ds eve RNA in the early blastoderm (4–5 h AEL). About 100% of the injected embryos share the same phenotype with eve RNA interference (RNAi) embryos generated through maternal RNAi [44] . Clones marked between 60 and 80% egg length in the RNAi embryos do not differ significantly from controls in the amount of cell division ( Fig. 2d ), but fail to elongate along the AP axis ( Fig. 2f ). Thus, as in Drosophila and consistent with the hypothesis of Benton et al . [40] , the cell rearrangements that drive elongation in the early Tribolium germband depend on eve function. Segments appear with a changing periodicity We found that the different degrees of cell rearrangement between anteriorly and posteriorly originating clones in Tribolium coincide with temporal heterogeneity in segment addition as measured throughout germband elongation. We analysed the rate of segment addition (as indicated by EN expression) throughout the entire period of germband extension. A linear regression through all time points yields an overall rate of segment addition of one segment added approximately every 45 min ( Supplementary Fig. 3 ). This is consistent with published rates calculated from shorter periods of segmentation [14] , [39] . However, when we analyse the temporal variation in segment addition throughout germband extension, we find a strikingly different pattern ( Fig. 3a ). Instead of a constant rate of segment addition, we find segments added in rapid bursts followed by slower rates of addition. This variability is most evident when comparing the change in segments added between 2-h time points: at about 16 h AEL, segment addition slows until 18 h AEL when there is a burst of five to six segments added over 2 h. This burst adds almost twice as many segments as during the 12–14-h and 14–16-h intervals and five times as many as during the 16–18-h interval ( Fig. 3b,c ). Segment addition in Tribolium is non-linear and calculating a single overall rate of segment addition masks the actual time course of segment addition, alternatively over and underestimating the actual rate. Furthermore, the abdominal segments formed during the rapid burst of segmentation are the same segments to which the dramatically elongated posterior clones contribute. Thus, there is likely a link between the spatial and temporal variability in thoracic versus abdominal germband development ( Supplementary Fig. 2 ). 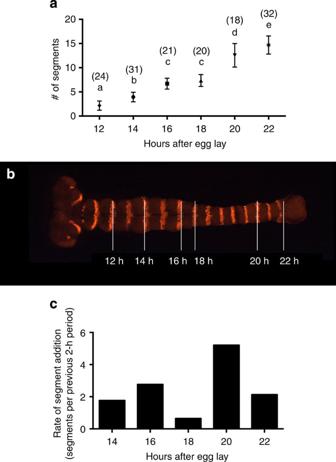Figure 3: Segment addition throughout germband elongation inTriboliumis not linear. To determine the rate of segment addition, we measured segment number at 2-h time intervals from 12 to 22 h AEL (embryos labelled, for example, 12 h could be 11 to 12 h since each egg lay was 1-h long). A linear regression through a scatter plot of all time points gave a segmentation rate of 1.3 segments per hour (seeSupplementary Fig. 3). However, analysing the variance between time intervals demonstrates that segment addition is not linear but is better characterized as having intervals of distinct periodicity (a, numbers in parentheses indicate group sample size; letters denote statistical significance; analysis of variance:R2=0.91,F=278; for replicates seeSupplementary Fig. 4). In particular, segment addition slows between 16 and 18 h, a time that roughly corresponds to the transition from adding thoracic to abdominal segments (b). This is followed by a rapid period of segment addition between 18 and 20 h. The direct comparison of rate of segment addition (c) clearly demonstrates that the period is not constant during germband elongation. Bars represent difference between averages of successive time points. Scale bar, 100 μm. Figure 3: Segment addition throughout germband elongation in Tribolium is not linear. To determine the rate of segment addition, we measured segment number at 2-h time intervals from 12 to 22 h AEL (embryos labelled, for example, 12 h could be 11 to 12 h since each egg lay was 1-h long). A linear regression through a scatter plot of all time points gave a segmentation rate of 1.3 segments per hour (see Supplementary Fig. 3 ). However, analysing the variance between time intervals demonstrates that segment addition is not linear but is better characterized as having intervals of distinct periodicity ( a , numbers in parentheses indicate group sample size; letters denote statistical significance; analysis of variance: R 2 =0.91, F =278; for replicates see Supplementary Fig. 4 ). In particular, segment addition slows between 16 and 18 h, a time that roughly corresponds to the transition from adding thoracic to abdominal segments ( b ). This is followed by a rapid period of segment addition between 18 and 20 h. The direct comparison of rate of segment addition ( c ) clearly demonstrates that the period is not constant during germband elongation. Bars represent difference between averages of successive time points. Scale bar, 100 μm. Full size image Abdominal segmentation can be simulated without cell division To explore whether the bulk of posterior elongation could occur without cell division, we modelled the 2-h window (18–20 h AEL) in which segment number increases from 7 to 12 segments. We built a computational model of the growth zone using the cell-based CompuCell3D simulation software ( compucell3d.org ) [45] . The initial conditions for our modelled growth zone were chosen to match the measured dimensions and cell counts in the growth zone in 18-h Tribolium embryos ( Fig. 4a,b ). Cells in the computational model do not divide. Rather they have both an intrinsic random motility and a position-dependent tendency to move in a particular direction that mimics cell trajectories observed in the earlier germband by Sarrazin et al . [14] Periodically, a new segment forms automatically at the anterior end of the modelled growth zone; each new segment is approximately eight cells long, reflecting measurements from embryos. Simulations of the model that produce five additional segments ( Fig. 4c ) produce elongated germbands and reduced growth zones similar to those in 20-h Tribolium embryos ( Fig. 4d ). While our computational model is simple—we have not attempted to model the mechanisms that drive cell rearrangements—it supports a model of germband elongation during abdominal segmentation that is driven primarily by cell rearrangement. Modelling growth zone dynamics using cell behaviours from specific species demonstrates that despite the default assumption of a posterior zone of higher mitotic activity, elongation can occur without localized posterior proliferation (see also [46] ). 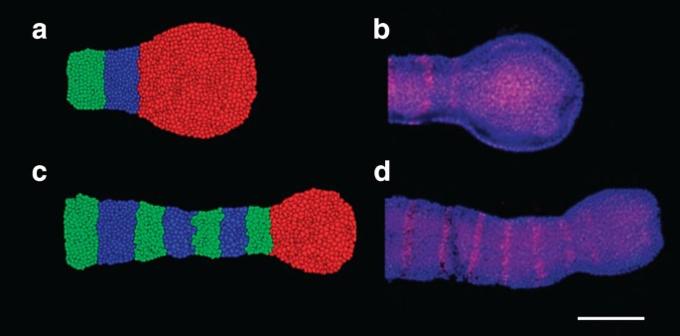Figure 4: Comparisons of the simulated and actualTriboliumgrowth zones. We built a computational model of growth zone elongation during the 18–20-h period of rapid segment addition inTribolium. Initial growth zone length and cell counts for the model (a) matched those measured in typical 18 h embryos (b). Elongation in the modelled growth zone depends on cell rearrangements (chosen to mimic those observed by Sarrazin,et al.14, in the earlierTriboliumembryo)—cells do not divide in the model. Over the modelled time window, the simulated germ band forms five additional segments (c), resembling the actual embryo (d). While we do not attempt to model the mechanisms leading to cell rearrangements or claim that cell rearrangements in the simulation exactly reflect those in the actual embryo, the simulation is consistent with a model in which cell rearrangements rather than a highly proliferative posterior growth zone drive axial elongation. Scale bar, 100 μm. Figure 4: Comparisons of the simulated and actual Tribolium growth zones. We built a computational model of growth zone elongation during the 18–20-h period of rapid segment addition in Tribolium . Initial growth zone length and cell counts for the model ( a ) matched those measured in typical 18 h embryos ( b ). Elongation in the modelled growth zone depends on cell rearrangements (chosen to mimic those observed by Sarrazin, et al . [14] , in the earlier Tribolium embryo)—cells do not divide in the model. Over the modelled time window, the simulated germ band forms five additional segments ( c ), resembling the actual embryo ( d ). While we do not attempt to model the mechanisms leading to cell rearrangements or claim that cell rearrangements in the simulation exactly reflect those in the actual embryo, the simulation is consistent with a model in which cell rearrangements rather than a highly proliferative posterior growth zone drive axial elongation. Scale bar, 100 μm. Full size image Our results contribute to an emerging view of the late blastoderm in Tribolium as consisting of highly motile cells that undergo only a small number of cell divisions to generate the elongated germband. We report for the first time that marked clones in the posterior blastoderm—the region fated to become the posterior growth zone in the elongating embryo—behave quite differently from anterior clones: posterior clones elongate more and give rise to a greater number of segments than anterior clones. This is not due to greater cell proliferation in the posterior: we find that anterior and posterior clones undergo the same modest amount of cell division, and that segment formation depletes cell numbers in the growth zone. Instead, the relatively extreme elongation of posterior clones is driven by considerably more cell rearrangement in the posterior ‘growth zone’ compared with the anterior region. Our computational model supports this view of posterior elongation driven primarily by cell rearrangement rather than cell proliferation. The idea that cells in the so-called growth zones of insect embryos might undergo cell rearrangement has long been suggested [26] , [29] , [30] , [31] , [47] , [48] , [49] , [50] but direct evidence was lacking, even in well-studied Tribolium embryos. Our data extend and refine two prior studies that suggest a significant role for cell movement in Tribolium germband elongation [14] , [40] . In a recent demonstration of cell rearrangement in the anterior blastoderm, Benton et al . [40] document adjacent cells interdigitating over a 1-h period. By contrast, our examination of ectodermal clones in the posterior blastoderm shows no evidence of cells having undergone multiple rounds of sliding intercalation. Instead, neighbouring cells and their progeny maintain contact as the embryo lengthens, even during extreme clonal elongation. Interestingly, mesodermal clones behave differently: marked mesodermal cells intercalate with unmarked cells (not shown). We conclude that, in Tribolium , the region commonly referred to as the ‘growth zone’ can best be viewed as distinguished primarily by cells of much higher motility, rather than as a proliferative pool of cells fuelling elongation. Classical categories of insect embryogenesis—short, intermediate and long germband–included the idea that there were differences in the number of segments inferred to be patterned in the blastoderm compared with those patterned in the growth zone [24] . In short germband embryos, procephalic and gnathal segments are patterned in the blastoderm, whereas in intermediate germband embryos thoracic and anterior abdominal segments are patterned in the blastoderm. Short of being able to transplant marked blastoderm cells to ectopic locations, however, the number of segments patterned in the blastoderm is challenging to determine experimentally. It has been thought that expression of segmentation genes might provide useful shorthand for determining which segments are patterned at the blastoderm. Tribolium blastoderm embryos, for instance, have two stripes of pair-rule gene expression, so it has been inferred that the gnathal and first thoracic segment are patterned in the blastoderm [30] . However, our data point to an apparent ambiguity when comparing segmental fates of marked blastoderm cells with pair-rule stripes. Cells at 60% EL in the early blastoderm can give rise to the second and third thoracic segments, which should arise from the third pair-rule stripe. However, the third pair-rule stripe first appears at the posterior tip of the embryo, as the posterior amniotic fold begins to form. This discrepancy highlights the dynamic nature of the blastoderm and the significant amount of rapid posterior movement blastoderm cells undergo. While our data do not provide a complete fate map of the Tribolium blastoderm, the clonal analysis also suggests that blastoderm cells are not yet restricted to individual segment identities since clones readily cross segmental boundaries. In general, our data demonstrate how clonal fates can provide another means to explore patterning present at the blastoderm stage. The boundary between blastoderm versus growth zone-patterned segments is a variable character in insect evolution; measurable discontinuities in clone behaviour may provide another means to characterize how this boundary is evolving. The spatial discontinuity in the behaviour of blastoderm clones correlates with an unexpected temporal discontinuity in segment addition. When we examine the rate of segment addition on a fine temporal scale—by comparing successive time points during germband elongation—segments form at strikingly variable rates. In the middle of germband extension, there is first a marked slowing in segment addition then a phase of rapid segment addition. This effect is hidden when average rates of segment addition are calculated for the entire period of germband elongation. In that case, we find that segments are added at a rate of one every 45 min (30 °C), an average rate is consistent with the previously published data (see also Supplementary Fig. 3 ): Sarazzin et al . [14] report about 95 min for each cycle of odd-skipped (a double segment period, 30 °C) and El-Sherif et al . [39] report similar average rates. Our data differ from these reports in that we track segment addition by following EN expression rather than pair-rule gene expression but the overall measured rate of segmentation is similar regardless of which marker is used. Of note, El-Sherif et al . [39] mention that the timing of the appearance of primary pair-rule stripes in the germband is on average shorter than those appearing in the blastoderm, and that the terminal pair-rule stripe is delayed in its appearance. However, whether that noted variation is similar to what we have observed with the appearance of En stripes remains to be determined. What is striking about both the spatial and temporal discontinuities we find, that is, the behaviour of clones and the rate of segment addition, is that both occur around the transition from thorax to abdomen during embryogenesis. The short anterior blastoderm clones form gnathal and thoracic segments and the long posterior blastoderm clones form abdominal segments. Similarly, the drop in segmentation rate occurs on average after the thorax is patterned and prior to a rapid burst of segment addition that adds abdominal segments. This suggests that the transition from thoracic to abdominal segments is an important regulatory boundary in Tribolium . Indeed, the pause in segment addition could be due to changes in underlying cellular mechanisms of growth and elongation, corresponding to the critical role that extensive cell rearrangements play during the phase of rapid abdominal segmentation. In a recent analysis of centipedes, temporal variation is linked to a switch between a mechanism that counts with a two segment periodicity to one which generates single segments [16] . Recently published work [51] suggests the terminal Tribolium segments may also switch from a pair-rule patterning mechanism to an unknown mechanism that generated single segments. Similarly, in a detailed analysis of axial variability in vertebrate segmentation, the transition between a constant rate of addition to a gradually slowing rate occurs at approximately the trunk/tail boundary [6] . The variability in segmentation rate we demonstrate in Tribolium forms a contrast to the regular segmental periodicity observed in the vertebrate trunk [6] . Within vertebrate species, the clock that drives segmentation for most of embryogenesis is very consistent, allowing researchers to describe species-specific periods. When it occurs, variation in the rate of segment addition tends to flank a longer phase of regular segment addition, for example, an early phase of rapid addition [7] or a slowing down of terminal segment addition [6] , [51] . Variants tend to be viewed in light of the more constant phase; slowing, for example, is thought to represent a gradual winding down of segmentation. The change in segmentation rate in Tribolium happens in the middle of segment addition and is striking in degree: less than one segment added over 2 h followed by five to six segments in the next 2 h. The lack of a single, monotonic rate of segment addition refutes the idea that segmentation in Tribolium is ‘clock like’ to the extent seen in vertebrates. Our data do not rule out oscillations as a patterning mechanism in the posterior, but they do suggest oscillations when measured throughout germband elongation are likely to vary in period. Alternatively there could be mismatch between the period of the clock and the rate of EN specification. Such a mismatch has recently been demonstrated in a vertebrate thought to have a relatively constant clock (zebrafish [53] ); there is a difference in period between the posterior oscillations in one of the clock genes (Hes1) and the anterior morphological formation of segments. However, the phenomena described there could not produce the kind of short/long/short-period variability we report here in Tribolium . In Tribolium , the orchestrated variability we document during elongation and segment addition suggests that neither a segmentation clock nor mechanisms of elongation are adequately captured by steady-state concepts. Instead, both appear dynamic and integrated by means we are yet to discover. Normal growth and segment addition To produce eggs cohorts of the same age, eggs were collected over a 1-h period from a mixed population of adults placed on white flour. The resulting cohorts of eggs of known birthdates were raised at 30 °C for specific durations, that is, 12, 14, 16, 18, 20, 22 h (AEL) measured from when the adults were added to the flour. Because eggs cannot be collected instantly, any age cohort can have animals up to an hour younger, for example, ‘12 h animals include animals from 11–12-h old. Handel et al . [54] claim that adults do not lay immediately on being transferred. If this is correct, the cohorts are likely to vary less than an hour in age and be biased towards the removal time, for example, 11–12-h animals are likely to be 11–11.75-h old. Embryos were fixed and stained with anti-EN (4D9; Developmental Studies Hybridoma Bank (DSHB)) and DAPI, and photographed on a Nikon E600 Ellipse epifluorescence microscope using a Spot digital camera (Diagnostics) and software. Number of EN stripes was scored in each individual and measures were taken to characterize the elongating germband. Note that rapid addition of segments between the 18–20-h time points means that animals at EN stages 10–13 were rarely sampled. Therefore, in the data presented in Fig. 1 , untimed animals at those developmental stages were added. All measurements were made directly on the photographs within the Spot software. In all images, the germband is peeled away from the yolk and the overlying serosa, and consists of two closely apposed epithelial layers—the ectoderm and the amnion, underlain by a progressively invaginating mesoderm. Measures treated the embryos as a two-dimensional sheet of epithelium and ingressed mesodermal cells were not quantified in any way. Measures were defined as follows (see Fig. 1e ): Germband length: line extending along the midline from between the two head lobes to the end of the germband (if the germband was bent, as in Fig. 1 , the length was measured as the sum of straight lines approximating the bend) Germband area: area measured from the mandibular EN stripe to the end of the germband (head lobes were excluded) Growth zone length: length along the midline from the last EN stripe to the end of the germband Growth zone area: area of region behind the last EN stripe Length of last segment: length along the midline between the last two EN stripes (that is, the most recently added segment) Area of last segment: area between the last two EN stripes All scatter plots with lines represent linear regressions of the data; all multiple comparisons are done by analysis of variance and show averages with s.d. Statistical analyses were performed using GraphPad Prism 6 software. Lineage tracing Embryos were collected over a 1-h period and cultured for 4 h (30 °C). Embryos were dechorionated (2% bleach solution for 2 min) and injected with caged fluorescein 4,5-dimethoxy-2-nitrobenzyl (DMNB-caged fluorescein; Invitrogen) and fluorescent dextran (fluoro-ruby; Molecular Probes) as a general cytoplasm marker that allowed for embryo staging. Embryos were cultured in M3+ insect medium [14] allowing the DMNB and dextran to diffuse throughout the syncytial blastoderm. Subsequent to injection, embryos were grown in M3+ insect medium [14] allowing the DMNB and dextran to diffuse throughout the syncytial blastoderm. Because it was not possible to maintain the embryos at 300C throughout the injection protocol, their developmental age could not be categorized by time after egg laying. Embryos were imaged at the time of injection to allow for subsequent determination of both total nuclei present and nuclear density to appropriately stage the embryos. Both of these values, when compared with embryos developing at constant temperature AEL, allowed us to determine the approximate age of the embryo at the time of marking the clone. At the time of activation, embryos corresponded to the stages labelled B1–B6 in the study by El-Sherif et al . [39] No evidence of serosal cells or the terminal primitive pit was present. Embryos marked at either earlier or later stages were not included in the present report. In interpreting the marked clones relative to published accounts of pair-rule gene expression patterns in the blastoderm [39] , it is important to note that cells in the blastoderm are motile [14] , [39] , [40] . They can either move towards the posterior or canroughly stay in the same position along the length of the embryo, depending on their dorsoventral position in the embryo. Based on the data in El-Sherif et al . [39] a blastoderm cell can move as much as 12% EL towards the posterior between an early blastoderm and a later blastoderm stage. Therefore, it is feasible that a clone marked in the blastoderm with an anterior border at 50% EL could be as far posterior as 62% EL at later blastoderm stages. DMNB was activated in a small cluster of cells using a × 40 objective lens and 405 nm ultraviolet light for a 30 s pulse on a Zeiss 510 confocal microscope. Embryos were cultured for variable lengths of time, fixed in 4% formaldehyde in PIPES, EDTA, Magnesium (PEM) buffer [55] and dissected by hand. Immunohistochemistry was performed with anti-EN (4D9; 25 μg ml −1 ; DSHB) and anti-fluorescein antibodies (Invitrogen; 1:100) to enhance the detection of the uncaged fluorescein. Embryos were imaged on both a Zeiss epifluorescence microscope and Zeiss 510 confocal microscope. All clones were analysed by confocal microscopy to determine which germ layer they contributed to. Only clones that contributed to the ectoderm are shown in Fig. 2 ; only clones that contribute to the ectoderm were included in our analysis of cell division rates. All clones, regardless of germ layer contribution were included in Supplementary Fig. 2 showing positional distribution. Image analyses of the cell lineage tracing experiments Cell counts and overall measurements were made on digitized images using NIH ImageJ. A total of 121 clones were scored; 6 measurements were taken on different sets of these embryos. (1) Anterior and posterior boundaries of the photo-activated area at the blastoderm stage were measured in relation to the total egg length. 0% corresponds to the anterior and 100% corresponds to the posterior end of the embryo, measured at its greatest length. (2) The number of segments each clone contributed to in the fully segmented germband with anti-EN antibody staining as a marker of the segmental boundaries. If a clone had only a very few cells (3–5) within a segment, it was not included. (3) The number of labelled cells at the blastoderm stage was counted using the cell counter tool on ImageJ, then checked by eye; (4) in the later stages, the labelled cells were counted using the ImageJ plug-in Image-based Tool for Counting Nuclei (ITCN). Z-stacks of images generated on the confocal were constructed using the specific slices in which labelled cells were detected. In the z-stack, labelled cells were carefully selected with polygon selection tool. The number of the nuclei detected with DAPI staining was counted in the same selected area. (5) The number of times cells within a clone divided was calculated based on the number of labelled cells immediately after DMNB photoactivation and at the endpoint of the experiment (later embryonic stages). (6) To measure the aspect ratio of the clones, labelled cells were selected with the polygon selection tool. The major axis (anteroposterior length) and minor axis (dorsoventral length) of the selected area were measured using the measurement tool. The aspect ratio was calculated as major axis/minor axis. The change of aspect ratio over time was calculated as aspect ratio at the endpoint/aspect ratio at time zero. All measurements were taken independently by three individuals, with an average of the three measurements used for each analysis. Eve RNAi Embryos were prepared as for lineage tracing. Double-stranded RNA was synthesized using an Ambion Megascript Kit; 500 bp eve clone. Embryos were injected at 4–5 h AEL with 100 ng μl −1 ds eve RNA, along with the DMNB and fluorescent dextran; n =16 embryos. ds eve RNA injected and buffer-injected controls were reared for 18–19 h (25 °C), when control embryos typically have 15 post-antennal EN stripes. The phenotypes mimicked published results using the same construct for pupal RNAi injections [44] . Modelling We simulated the developing 18–20 h Tribolium germ band using the CompuCell3D simulation environment (available for download at compucell3d.org). CompuCell3D is an open-source software package that simulates multi-cell interactions and behaviours according to the Glazier–Graner–Hogeweg (GGH) model of cell behaviours [56] , [57] . For a more complete introduction to GGH modelling with CompuCell3D, see Swat et al . [57] See Supplementary Note 1 for additional details of the modelling. How to cite this article: Nakamoto, A. et al . Changing cell behaviours during beetle embryogenesis correlates with slowing of segmentation. Nat. Commun. 6:6635 doi: 10.1038/ncomms7635 (2015).